Ligand-controlled stereodivergent alkenylation of alkynes to access functionalizedtrans- andcis-1,3-dienes Precise stereocontrol of functionalized alkenes represents a long-standing research topic in organic synthesis. Nevertheless, the development of a catalytic, easily tunable synthetic approach for the stereodivergent synthesis of both E -selective and even more challenging Z -selective highly substituted 1,3-dienes from common substrates remains underexploited. Here, we report a photoredox and nickel dual catalytic strategy for the stereodivergent sulfonylalkenylation of terminal alkynes with vinyl triflates and sodium sulfinates under mild conditions. With a judicious choice of simple nickel catalyst and ligand, this method enables efficient and divergent access to both Z- and E- sulfonyl-1,3-dienes from the same set of simple starting materials. This method features broad substrate scope, good functional compatibility, and excellent chemo-, regio-, and stereoselectivity. Experimental and DFT mechanistic studies offer insights into the observed divergent stereoselectivity controlled by ligands. 1,3-Dienes are one of the most important structural motifs frequently found in many natural products and biologically active compounds [1] , [2] , as well as serve as valuable building blocks for diverse transformations in organic synthesis [3] , [4] . Accordingly, the stereoselective synthesis of 1,3-dienes has received paramount attention in organic synthesis [5] , [6] , [7] . Olefinations of carbonyls are widely embraced methods to access 1,3-dienes, while typically leading to E / Z isomers [8] , [9] . Alternatively, transition-metal-catalyzed cross-coupling reactions, including Heck couplings [10] , ene-yne couplings [11] , hydrovinylation of alkynes [12] , alkenyl-alkenyl couplings [13] , [14] , [15] , and boroalkenylation of alkynes [16] , [17] , [18] , [19] , have emerged as a powerful strategy for the stereoselective synthesis of 1,3-dienes. Despite enabling, these methods generally lead to thermodynamically more stable E -isomers, or rely on the use of stereochemically well-defined organometallic agents or electrophiles. To the best of our knowledge, catalytic stereodivergent protocol that would enable both E -selective and even more challenging Z -selective access of highly substituted 1,3-dienes from one set of substrates remains underexploited [20] , [21] . Ni-catalyzed vicinal difunctionalization of alkynes via metalation followed by subsequent functionalization of alkenyl nickel species represents an attractive strategy for the synthesis of substituted alkenes from simple starting materials [22] , [23] , [24] , [25] , [26] . The highly stereoselective metalation step ensures the selective construction of syn -addition products, with a few exceptions of anti -selective examples that proceed via substrate-driving E/Z isomerization of alkenyl nickel species [27] , [28] , [29] , [30] , [31] , [32] , [33] , [34] . Recently, radical-involved catalytic 1,2-difunctionalization of alkynes has been disclosed to furnish trisubstituted alkenes with complementary anti -selectivity [35] , [36] , [37] , [38] , [39] , [40] , [41] , [42] . Particularly, utilizing dual nickel/photoredox catalysis [43] , [44] , [45] , [46] , [47] has further exploited a number of selective difunctionalization of alkynes with diverse coupling partners under mild conditions [48] , [49] , [50] , [51] , [52] , [53] , [54] , [55] , [56] . Nevertheless, rare examples for stereodivergent synthesis of both trans - and cis -substituted alkenes from alkynes are reported. Recently, we reported a photoredox/nickel dual catalyzed stereodivergent difunctionalization of alkynes, furnishing both syn - and anti -selective aryl-substituted alkenes via the judicious choice of photocatalysts with different triplet state energies (Fig. 1a ) [57] . Despite attractive, such a contra -thermodynamic alkene isomerization strategy relies on the structure of alkenes or photocatalysts. Thus, the development of photoredox/nickel dual-catalyzed divergent method with a complementary stereoselective tuning strategy to access more diverse types of alkenes, such as functionalized cis- and trans -1,3-dienes, under mild and operationally simple conditions would be of particular interest. Fig. 1: Background and recent work of carbosulfonylation of alkynes. a Previous work: photocatalyst-controlled stereodivergent sulfonylarylation of alkynes. b This work: ligand-controlled stereodivergent alkenylation of alkynes to access functionalized 1,3-dienes. PC photocatalyst, EnT energy transfer, dppf 1,1-bis(diphenylphosphino)ferrocene, phen 1,10-phenanthroline. Full size image Here, we show a ligand-controlled stereodivergent alkenyl-functionalization of alkynes with vinyl triflates and sodium sulfinates via photoredox and nickel dual catalysis (Fig. 1b ). This strategy furnishes a wide array of synthetically valuable cis - and trans -sulfonyl-1,3-dienes [58] , [59] in one pot from simple starting materials. Detailed mechanistic experiments and computational investigations offer insights into the origins of the observed stereoselectivity and the role of dynamic ligand exchange in the dual ligand system. 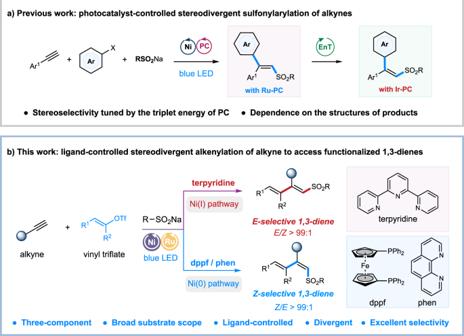Fig. 1: Background and recent work of carbosulfonylation of alkynes. aPrevious work: photocatalyst-controlled stereodivergent sulfonylarylation of alkynes.bThis work: ligand-controlled stereodivergent alkenylation of alkynes to access functionalized 1,3-dienes. PC photocatalyst, EnT energy transfer, dppf 1,1-bis(diphenylphosphino)ferrocene, phen 1,10-phenanthroline. Reaction optimizations Our investigations were started with phenylacetylene 1 , vinyl triflate 2 , and sodium p -tolylsulfinate 3 as model substrates (Table 1 ). After some experimentations, we found that in the presence of Ru(dtbbpy) 3 (PF 6 ) 2 as the photocatalyst, Ni(OAc) 2 •4H 2 O as the nickel catalyst, and 1,10-phenanthroline (1,10-phen) as the ligand, irradiation of the reaction mixture in DMF with blue LEDs gave the sulfonylated diene product 4b in 45% yield with excellent regio- and anti -selectivity (entry 1). Pleasingly, employing terpyridine (tpy) as the ligand dramatically improved the yield of product 4b to 86% without observation of syn -selective isomer (entry 2). Further evaluation of nickel catalysts or pre-catalysts disclosed that Ni(OAc) 2 •4H 2 O was the optimal catalyst for this anti- selective transformation (entries 3-6). During this process, we noticed that the nature of nickel salts played an intriguing effect on the trans/cis selectivity. Switching to phosphine-ligated nickel pre-catalysts resulted in the formation of a mixture of trans/cis isomers 4a and 4b in varied yields and Z/E ratios (entries 4–6). Interestingly, the use of NiCl 2 •dppf in the absence of terpyridine led to the exclusive formation of syn -selective product 4a , albeit in low yield (entry 7). The addition of 1,10-phen as an exogenous ligand turned out to be beneficial to the yield of 4b , together with the formation of isomer 4a (entry 8) [60] . Careful examination of the ratio of nickel and ligand revealed that the use of 20 mol% NiCl 2 •dppf with 10 mol% 1,10-phen furnished 4a in 80% yield with excellent cis/trans selectivity (entries 8–11). Finally, control experiments disclosed that photocatalyst, nickel catalyst, and light were all essential for this stereodivergent reaction (entries 12–14) (see Supplementary Information for more optimization details). Table 1 Optimization of reaction conditions a Full size table Substrate scope studies With the optimal reaction conditions in hand, we began to investigate the substrate compatibility of this stereodivergent protocol in the presence of Ru(dtbbpy) 3 (PF 6 ) 2 with two sets of nickel catalysts (entries 2 and 11, respectively). As shown in Fig. 2 , a series of cyclic vinyl triflates smoothly underwent cross-couplings with phenyl acetylene 1 and TsNa 3 , furnishing 1,3-dienyl sulfones with high efficiency and excellent Z or E -selectivity ( 4a – 18a & 4b – 18b ). Cyclohexenyl triflates with substituents on 4-position, including alkyl, aryl, ketal, and ester, were well compatible; interestingly, ortho -substituents turned out to be well-tolerated with any deleterious effect to the coupling yield and cis/trans selectivity ( 10a & 10b ). Moreover, vinyl triflates derived from heteroatom-incorporated cyclic ketones, represented by tetrahydro-4 H -pyran-4-one and 4-piperidinone, were competent coupling partners, affording corresponding dienes with excellent selectivity ( 12a – 13a & 12b – 13b ). The reaction of cyclic vinyl triflates that were prepared from 5-, 7- and 8-membered cyclic ketones proceeded smoothly, albeit with slightly decreased E/Z selectivity in the case of 5-membered vinyl triflate ( 14a – 17a & 14b – 17b ). Pleasingly, acyclic vinyl triflates that derived from aliphatic ketones were suitable substrates, furnishing the diene products with excellent selectivity yet decreased yields ( 18a-21a & 18b-21b ). The reactions with 1,2-disubstituted vinyl triflates produced the desired coupling products with excellent syn- selectivity yet low anti- selectivity ( 22a & 22b ). It should be noted that the structures of products 13a and 13b are validated by single-crystal X-ray diffraction and the stereoselectivity of the two isomers of products 4a & 4b , 13 & 13b , 22a & 22b , 25a & 25b , and 53a & 53b is further confirmed by COSEY and NOSEY. The stereoselectivity of other products is assigned by analogy. Fig. 2: Substrate Scope. Reaction conditions: Ru(dtbbpy) 3 (PF 6 ) 2 (1 mol%), Ni(OAc) 2 •4H 2 O/tpy (for anti -selective), NiCl 2 •dppf/1,10-phen (for syn -selective), alkyne (1.5 equiv. ), vinyl triflate (0.1 mmol), sodium sulfinate (1.5 equiv. ), DMF [0.04 M], 35 o C, blue LED, 6 h. Isolated yields. Ts = toluenesulfonyl. Full size image Next, we turned our attention to the scope of the alkyne component (Fig. 2 ). A wide range of aryl alkynes, bearing electron-donating or withdrawing substituents on the ortho- , meta -, or para -positions of aromatic rings, all underwent efficient couplings to furnish sulfonated 1,3-dienes with excellent stereoselectivity ( 23a – 37a & 23b – 37b ). The mild conditions were compatible with diverse functional groups, including esters, halides, phenols, and amines, leaving synthetic handles for further potential manipulations. Acetylenes incorporated with a heteroarene, represented by quinoline, thiophene, and dibenzo[ b,d ]furan, all worked well with high efficiency ( 35a – 36a, 38a & 35b – 36b, 38b ). 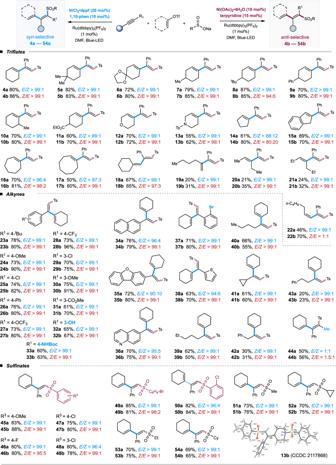Fig. 2: Substrate Scope. Reaction conditions: Ru(dtbbpy)3(PF6)2(1 mol%), Ni(OAc)2•4H2O/tpy (foranti-selective), NiCl2•dppf/1,10-phen (forsyn-selective), alkyne (1.5 equiv.), vinyl triflate (0.1 mmol), sodium sulfinate (1.5 equiv.), DMF [0.04 M], 35oC, blue LED, 6 h. Isolated yields. Ts = toluenesulfonyl. 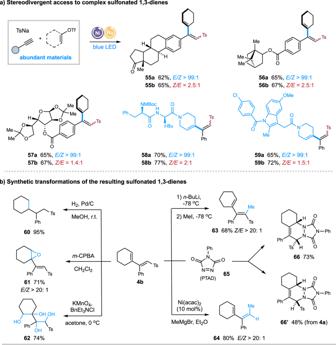Fig. 3: Synthetic applications. aStereodivergent access to complex sulfonyl 1,3-dienes;bSynthetic transformations of sulfonyl 1,3-dienes.m-CPBA =m-chloroperoxybenzoic acid. Besides, aliphatic terminal alkynes were suitable substrates, affording functionalized 1,3-dienes in decreased yields yet with excellent Z / E selectivity ( 39a – 43a & 39b – 43b ). Nevertheless, the reaction of internal alkynes only proceeded with moderate trans/cis selectivity under these two reaction conditions ( 44a & 44b ). Last, a number of sodium alkyl sulfinates and substituted aryl sulfinates all participated in the dual catalytic divergent protocol smoothly, delivering the desired sulfonyl-1,3-diene products with high yields and excellent regio- and syn/anti -selectivity ( 45a – 54a & 45b – 54b ). To further demonstrate the synthetic applicability of this dual-protocol, late-stage modifications of complex molecules have been evaluated (Fig. 3a ). 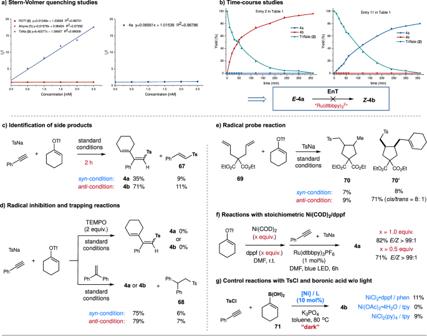Fig. 4: Mechanistic studies. aStern-Volmer quenching studies;bTime-course studies;cIdentification of side products;dRadical inhibition and trapping reactions;eRadical probe reaction;fReaction with stoichiometric Ni(COD)2/dppf;gControl reactions with TsCl and boronic acid w/o light. EnT = Energy transfer. Under the syn -selective conditions (entry 11, Table 1 ), the reaction of complex terminal alkynes or vinyl triflates, derived from estrone, indomethacin (anti-inflammatory), glucose, borneol, and amino acid, proceeded smoothly to afford the desired E -1,3-dienes with high yields and excellent stereoselectivity ( 55a – 59a ). Under the anti -selective condition (entry 2, Table 1 ), nevertheless, reactions with these complex substrates proceeded in comparable yields yet moderate stereoselectivity, probably due to the significant steric hindrance of these complex substrates ( 55b – 59b ). Moreover, the resulting sulfonyl 1,3-dienes are useful building blocks in organic synthesis (Fig. 3b ). Hydrogenation of 4b in the presence of palladium on carbon (Pd/C) and H 2 gave alkyl sulfone 60 in 95% yield. 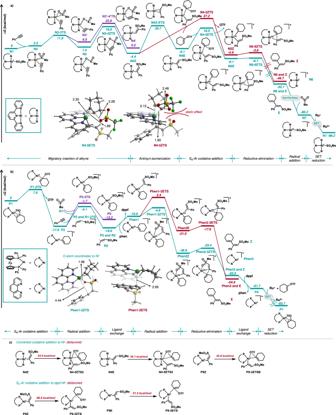Fig. 5: DFT calculations. aDFT-computed energy profiles for the sulfonylalkenylation with terpyridine ligand.bDFT-computed energy profiles for the sulfonylalkenylation with dppf and phenanthroline ligand.cEnergy barriers of concerted oxidative addition to NiIand SN-Ar oxidative addition to NiIwith dppf ligand. Free energies in solution (in kcal·mol-1) were calculated at SMD (DMF)-M06/Def2-TZVPP//PBE-D3(BJ)/Def2-TZVP (Ni, Fe, Ru)/Def2-SVP (other atoms). DFT-optimized geometries of selected transition states or intermediates are shown. Bond lengths are in Å. Oxidation of 4b with m -CPBA or KMnO 4 yielded epoxide 61 and polyol 62 , respectively. Furthermore, treatment of 4b with n -butyllithium, followed by the addition of MeI, afforded 68% yield of ( Z )-tetra-substituted sulfonyl alkene 63 , the stereoselective synthesis of which remains challenging. Cross-coupling of 4b with methylmagnesium bromide in the presence of catalytic Ni(acac) 2 furnished ( E )-tri-substituted 1,3-dienes 64 in 78% yield and excellent stereoselectivity. Finally, cycloaddition reactions of 4a or 4b with 4-phenyl-1,2,4-triazoline-3,5-dione (PTAD) 65 resulted in the formation of the two stereoisomers of products 66 and 66’ in moderate yields. Fig. 3: Synthetic applications. a Stereodivergent access to complex sulfonyl 1,3-dienes; b Synthetic transformations of sulfonyl 1,3-dienes. m -CPBA = m -chloroperoxybenzoic acid. Full size image Mechanistic studies To gain insights into the potential mechanism, we have performed some preliminary mechanistic experiments (Fig. 4 ). On the one hand, we conducted a number of experiments regarding the photocatalytic part. Stern-Volmer fluorescence quenching studies indicated that the photoexcited *Ru(dtbbpy) 3 2+ was quenched by TsNa, other than alkyne 1 or vinyl triflate 2 (Fig. 4a ). 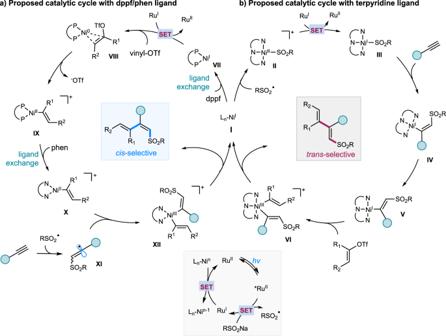Fig. 6: Proposed reaction pathways. aProposed catalytic cycle with dppf/phen ligand.bProposed catalytic cycle with terpydine ligand. dppf = 1,1-bis(diphenylphosphino)ferrocene; phen = 1,10-phenanthroline.hv= visible light. SET = single electron transfer. Light on/off experiments under both anti - and syn- selective conditions were performed, which showed that the desired couplings ceased in the dark (See Supplementary Figure 6 – 7 ); additionally, quantum yields (ϕ) of both anti - and syn -selective reactions were determined to be less than 1 (See Supplementary Information) [61] . These results ruled out the possibility of a radical chain pathway in this photochemical process. Furthermore, time-course studies of template reactions (phenylacetylene 1 , vinyl triflate 2 , and TsNa 3 ) showed that anti/syn -selectivity of products 4a and 4b remained steady under the conditions shown in entries 2 or 11 (Fig. 4b ). Additionally, no significant fluorescence quenching effect was observed between E - 4a and photoexcited *Ru(dtbbpy) 3 2+ (E T ≈ 46 kcal/mol) [57] (Fig. 4a ). These results precluded the involvement of photocatalytic E → Z isomerization of sulfonyl 1,3-dienes, thus further supporting ligand control of stereoselectivity in this catalytic system [57] . On the other hand, we detected a small amount of side product E -51 with careful monitoring of this reaction, implying that this reaction could proceed via sulfonyl addition followed by alkenylation (Fig. 4c ). Then, radical inhibition and probe reactions were performed (Figs. 4 d- 4e ). The addition of 2,2,6,6-tetramethyl-1-piperidinyloxy (TEMPO) into the standard systems (entries 1 and 11, Table 1 ) completely shut down the desired reactions, while the addition of 1,1-diphenylethylene gave the desired products 4a / 4b in slightly decreased yields, together with a small amount of alkyl sulfone adduct 68 (Fig. 4d ). Reaction of vinyl triflate 2 and TsNa with 1,5-diene 69 , instead of alkyne 1 , gave a small amount of tosylation/cyclization product 70 and tosylation/cyclization/alkenylation product 70’ under the syn -selective condition; interestingly, the parallel reaction under the anti -selective condition resulted in the formation of 9% yield of 70 , together with 71% yield of 70’ (Fig. 4e ). These results implied that different reaction pathways could be involved in syn- and anti- selective systems. Additionally, control reactions with stoichiometric Ni(cod) 2 and dppf in the absence of 1,10-phen gave good yields of product 4a ( Z/E > 99:1), in contrast to the results with catalytic Ni(cod) 2 /dppf (entry 7, Table 1 ), suggesting the importance of a synergistic effect with the two ligands (Fig. 4e ) [62] . Furthermore, the reaction of alkyne 1 , alkenyl boronic acid 71 , and TsCl with catalytic NiCl 2 (py) 4 /tpy or NiCl 2 •dppf/phen gave a small amount of anti -selective diene 4b under thermal conditions [35] , demonstrating the intriguing role of light irradiation in this stereodivergent alkenylation and further highlighting the synthetic advantage of this photochemical dual-protocol. Fig. 4: Mechanistic studies. a Stern-Volmer quenching studies; b Time-course studies; c Identification of side products; d Radical inhibition and trapping reactions; e Radical probe reaction; f Reaction with stoichiometric Ni(COD) 2 /dppf; g Control reactions with TsCl and boronic acid w/o light. EnT = Energy transfer. Full size image Next, we performed density functional theory (DFT) calculations to gain a deeper understanding of the mechanism and catalytic cycle, particularly to rationalize the stereoselectivity controlled by the different ligands (Computational details are given in the supporting information) (Fig. 5 ). We chose 51a / b as the model substrate with terpyridine and dppf/phenanthroline as the model ligands for the anti / syn selective conditions, respectively (Table 1 , entries 3 and 11). In Fig. 5a , the Ni-catalytic cycle with terpyridine as the ligand begins with the Ni I -SO 2 Me intermediate N1 [57] . First, phenylacetylene 1 coordinates to the intermediate N1 and produces N2 , followed by the rearrangement of the SO 2 Me moiety from a Ni-S to Ni-O bonding mode with an energy barrier of 11.9 kcal/mol ( N2-3TS ). Two intermediates are formed in which the sulfonyl group is in a suitable orientation to either attack the terminal ( N3 ) or internal ( N3’ ) carbon of the alkyne. The sulfonyl group then migrates to the terminal carbon of the alkyne via a five-membered ring transition state ( N3-4ZTS ) with an energy barrier of 18.4 kcal/mol. In contrast, the migratory insertion into the internal carbon is disfavored by 3.0 kcal/mol ( N3’-4’TS ), which is consistent with the observed regioselectivity of this reaction. In the intermediate N4Z , the phenyl and sulfonyl moieties are anti -oriented after migratory insertion. Thus, it can either undergo direct S N -Ar type of oxidative addition of vinyl triflate 2 via transition state N4-5ZTS , with an energy barrier of 31.6 kcal/mol, resulting in the syn -selective product 51b , or undergo anti / syn isomerization followed by oxidative addition. The C-C bond rotates during the anti / syn isomerization with an activation energy of 25.1 kcal/mol, leading to the intermediate N4E . The S N -Ar-type oxidative addition of vinyl triflate to N4E has an energy barrier of only 18.6 kcal/mol ( N4-5ETS ), which lies 8.7 kcal/mol below the transition state N4-5ZTS . The proximity of the sulfonyl and OTf groups in the transition state N4-5ZTS may account for the high oxidative addition energy barrier. A comparison of the two oxidative addition routes implies that the formation of anti -selective product E is preferred since the transition state N4Z-ETS is favored by 6.5 kcal/mol over N4-5ZTS , which explains the anti -stereoselectivity when terpyridine was used as the ligand. After the reductive elimination, the cross-coupling product is formed, together with the generation of the Ni I intermediate N6 . The reduction of N6 to Ni 0 intermediate N8 by the Ru-photocatalyst is calculated to be thermodynamically disfavored (+2.2 kcal/mol, see Supplementary Figure 19 ). In contrast, the radical addition of sulfonyl radical to N6 is barrierless, with an energy gain of 28.1 kcal/mol [63] , [64] . The generated Ni II intermediate N7 can then be reduced by the Ru-photocatalyst and start the next catalytic cycle. Fig. 5: DFT calculations. a DFT-computed energy profiles for the sulfonylalkenylation with terpyridine ligand. b DFT-computed energy profiles for the sulfonylalkenylation with dppf and phenanthroline ligand. c Energy barriers of concerted oxidative addition to Ni I and S N -Ar oxidative addition to Ni I with dppf ligand. Free energies in solution (in kcal·mol -1 ) were calculated at SMD (DMF)-M06/Def2-TZVPP//PBE-D3(BJ)/Def2-TZVP (Ni, Fe, Ru)/Def2-SVP (other atoms). DFT-optimized geometries of selected transition states or intermediates are shown. Bond lengths are in Å. Full size image Subsequently, the reaction with a dual ligand system (dppf and phenanthroline) was explored, and the catalytic cycle is depicted in Fig. 5b . Based on a recent report [62] , we proposed that the dynamic ligand exchanges on Ni intermediates promote different steps in the syn -selective catalytic cycle. The phosphine ligand dppf facilitates the Ni I reduction and Ni 0 oxidative addition steps, while the phenanthroline ligand facilitates the radical addition step. The binding of vinyl triflate 2 to dppf-Ni 0 forms the intermediate P1 , which undergoes S N -Ar-type oxidative addition to afford the Ni II cation P2 with an energy barrier of only 7.9 kcal/mol [65] , [66] . Next, the sulfonyl radical R1 can either add to P2 via the transition state P2-5TS with a 16.2 kcal/mol barrier, leading to P5 , or add to the alkyne, forming the vinyl radical R2 , with a barrier of 13.8 kcal/mol. The radical addition to an alkyne is kinetically and thermodynamically favored. The Ni II cation P2 then undergoes ligand exchange with phenanthroline to afford Ni II intermediate Phen1 . The vinyl radical R2 undergoes radical addition with two distinct orientations to the Ni II cation Phen1 , resulting in an anti- or syn- selective Ni III intermediate ( Phen2E or Phen2Z ). The transition state of the syn -selective radical addition is 14.1 kcal/mol (Phen1-2ZTS ), favored by 7.3 kcal/mol over the anti -selective radical addition ( Phen1-2ETS ), which may be due to the coordination of the oxygen atom from the sulfonyl group to the Ni II metal center. Also, the syn -selective Ni III intermediate Phen2Z is more stable than the anti -selective Ni III intermediate Phen2E (15.9 kcal/mol difference in energy). With a barrier of only 3.5 kcal/mol, the reductive elimination of Phen2Z is rapid, yielding the syn -selective product. The resulting Ni I cation Phen3 again undergoes ligand exchange with dppf to afford the dppf-Ni I intermediate P4 . In contrast to the tpy-Ni I intermediate N6 , the intermediate P4 can easily be reduced by the Ru-photocatalyst, leading to the formation of Ni 0 intermediate P1 with an energy gain of 32.0 kcal/mol. The concerted oxidative addition to Ni I intermediate via a three-membered ring transition state was calculated to be disfavored. In addition, the S N -Ar type oxidative addition to the dppf-Ni I intermediate is not feasible at room temperature for both anti - and syn -selective pathways (Fig. 5c ). Given that 32% syn -selective product was obtained when only dppf was used as the ligand (see Table 1 , entry 7), the syn -selective catalytic cycle with only dppf as the ligand was also explored (see Supplementary Figure 15 for the energy profile). The stereoselectivity can also be explained by the 19.1 kcal/mol energy difference between the anti/syn radical addition step ( P2-3ZTS vs . P2-3ETS ). Alternatively, another catalytic pathway involving the migratory insertion of alkyne to dppf-ligated vinyl-Ni species was investigated, in which the regio- and stereoselectivity can also be explained (See Supplementary Figure 16 for the energy profile). However, this pathway was not chosen as the main catalytic pathway due to the observed hydrosulfonylation by-product 51 (Fig. 4c ), which cannot be generated by this pathway. Based on these experimental and computational results, we propose a plausible reaction pathway as depicted in Fig. 6 . Upon light excitation, photoexcited *Ru(dtbbpy) 3 2+ ( E 1/2 *ox = +0.81 V vs. SCE) [67] , [68] interacts with RSO 2 Na (TsNa, E red = + 0.45 V versus SCE in CH 3 CN) [69] to release sulfonyl radical and the reducing Ru(I). In the case of terpyridine as ligand, the sulfonyl radical is trapped by Ni(I) I to give RSO 2 -Ni(II) II [57] , which is then single-electron reduced by Ru(I) to generate RSO 2 -Ni(I) II . Migratory insertion of II into alkyne III regioselectively delivers cis -alkenylNi(I) species IV , followed by isomerization, to afford the trans -alkenylNi(I) V . S N -Ar type oxidative addition of V with vinyl triflate affords trans -Ni(III) VI , followed by reductive elimination, to furnish anti -addition dienes. In the case of NiCl 2 •dppf/phen, which is more electron-rich and less sterically hindered compared to NiCl 2 (py) 4 /tpy, dppf-ligated Ni(I) VII is more prone to a SET reduction by Ru(I) to generate Ni(0) species, followed by binding and facile S N -Ar type oxidative addition with vinyl triflate to form dppf-ligated alkenylNi(II) IX . Then, IX undergoes ligand exchange with 1,10-phen to form phen-ligated alkenylNi(II) X . At the same time, the sulfonyl radical adds to alkyne to form vinyl radical XI , which is subsequently captured by phen-ligated alkenylNi(II) X to generate the more stable cis -Ni(III) species XII . Reductive elimination of Ni(III) XII furnishes syn -selective product as well as Ni(I) I , the latter of which undergoes ligand exchange with dppf to yield (dppf)Ni(I) VII . Finally, Ru(I) (Ru(dtbbpy) 3 + , E 1/2 II/I = −1.45 V vs SCE) [67] is feasible to reduce (dppf)Ni(I) VII or (terpy)Ni(II) II [ E 1/2 (Ni II /Ni 0 ) = −1.2 V versus SCE in DMF] [70] to regenerate the ground state Ru(dtbbpy) 3 2+ and close the two catalytic cycles. Fig. 6: Proposed reaction pathways. a Proposed catalytic cycle with dppf/phen ligand. b Proposed catalytic cycle with terpydine ligand. dppf = 1,1-bis(diphenylphosphino)ferrocene; phen = 1,10-phenanthroline. hv = visible light. SET = single electron transfer. Full size image In summary, we have developed a dual photoredox and nickel catalyzed stereodivergent three-component alkenyl-functionalization of alkynes with vinyl triflates and sodium sulfinates under mild and operationally simple conditions. Such a photochemical dual strategy enables divergent and straightforward access to syn- and anti -selective sulfonyl-1,3-dienes by a simple choice of nickel catalyst and ligand without the reliance on the structures of photocatalyst and alkene products. This method demonstrates broad substrate scope and excellent chemo-, regio-, and stereo-selectivity, with potential applications in late-stage functionalizations. A series of mechanistic experiments, including Stern-Volmer fluorescence quenching studies, light on/off experiments, determination of quantum yields, radical probe reactions, and time course studies, as well as detailed computational investigations, offer insights into the origins of the observed stereoselectivity controlled by simple ligands. General procedure for the cis-selective alkenylation To a flame-dried 8 mL reaction vial equipped with a magnetic stir bar was charged with Ru(dtbbpy) 3 (PF 6 ) 2 (1 mol %), NiCl 2 •dppf (20 mol %), 1,10-phenanthrane (10 mol %), sulfinate (1.5 equiv. ), and DMF [0.04 M]. The reaction mixture was degassed by nitrogen sparging for 30 min, followed by the addition of vinyl triflate (0.10 mmol) and alkyne (1.5 equiv). The reaction mixture was irradiated with blue LEDs for 6 h (around 35 °C, with a cooling fan placed on the top of the vial). The reaction mixture was quenched with water and extracted with ethyl acetate. The combined organic layers were dried with MgSO 4 , filtered and concentrated in vacuo. The crude material was purified by flash chromatography (silica gel, petroleum ether/ ethyl acetate) to afford the products. General procedures for the trans-selective alkenylation To a flame-dried 8 mL reaction vial equipped with a magnetic stir bar was charged with Ru(dtbbpy) 3 (PF 6 ) 2 (1 mol %), Ni(OAc) 2 • 4H 2 O (10 mol %), terpyridine (10 mol %), sulfinate (1.5 equiv.) and DMF [0.04 M]. The reaction mixture was degassed by nitrogen sparging for 30 min, followed by the addition of vinyl triflate (0.10 mmol) and alkyne (1.5 equiv.). Then the reaction mixture was irradiated with blue LEDs for 6 h (around 35 °C). The reaction mixture was quenched with water and extracted with ethyl acetate. The combined organic layers were dried with MgSO 4 , filtered and concentrated in vacuo. The crude material was purified by flash chromatography (silica gel, petroleum ether/ ethyl acetate) to afford the products.